miR-196b directly targets bothHOXA9/MEIS1oncogenes andFAStumour suppressor inMLL-rearranged leukaemia HOXA9 and MEIS1 have essential oncogenic roles in mixed lineage leukaemia ( MLL )-rearranged leukaemia. Here we show that they are direct targets of miRNA-196b, a microRNA (miRNA) located adjacent to and co-expressed with HOXA9 , in MLL -rearranged leukaemic cells. Forced expression of miR-196b significantly delays MLL -fusion-mediated leukemogenesis in primary bone marrow transplantation through suppressing Hoxa9 / Meis1 expression. However, ectopic expression of miR-196b results in more aggressive leukaemic phenotypes and causes much faster leukemogenesis in secondary transplantation than MLL fusion alone, likely through the further repression of Fas expression, a proapoptotic gene downregulated in MLL -rearranged leukaemia. Overexpression of FAS significantly inhibits leukemogenesis and reverses miR-196b-mediated phenotypes. Targeting Hoxa9/Meis1 and Fas by miR-196b is probably also important for normal haematopoiesis. Thus, our results uncover a previously unappreciated miRNA-regulation mechanism by which a single miRNA may target both oncogenes and tumour suppressors, simultaneously, or, sequentially, in tumourigenesis and normal development per cell differentiation, indicating that miRNA regulation is much more complex than previously thought. Human mixed lineage leukaemia ( MLL , HRX and ALL-1 ) gene, located at chromosome band 11q23, is involved in chromosomal translocations with over 60 different partner genes (for example, AF4 , AF6 , AF9 , AF10 , ELL and ENL ) in ∼ 10% of acute (myeloid or lymphoid) leukaemias, which are associated with unfavourable survival [1] , [2] . The resulting MLL fusion proteins transform cells primarily through direct upregulation of A-cluster HOX genes and HOX cofactors such as MEIS1 [3] , [4] , [5] , [6] , [7] , [8] , [9] . The mammalian HOX genes encode DNA-binding homeobox proteins that have a critical role in embryogenesis and haematopoiesis. MEIS1 is a homeodomain protein that acts as a DNA-binding cofactor of HOX proteins. HOXA and MEIS1 genes are normally expressed in haematopoietic progenitor cells and downregulated during differentiation [10] , [11] , [12] . Aberrant overexpression of HOXA and MEIS1 genes is a hallmark of MLL -rearranged leukaemia [3] , [13] , [14] . HOXA9 and MEIS1 have been shown to be the most critical downstream targets of MLL fusion proteins, and their coexpression is sufficient to transform cells and induce acute myeloid leukaemia (AML) [3] , [4] , [5] , [15] , [16] , [17] . Their aberrant overexpression has been shown to be required for the induction and maintenance of MLL -rearranged leukaemia [5] , [6] , [7] , [8] , [9] . MicroRNAs (miRNAs) are a class of small regulatory RNAs that bind directly to complementary sequences (usually at 3′-untranslated regions; that is, 3′ UTRs) on target messenger RNA (mRNA) transcripts, resulting in translational repression and/or target mRNA degradation [18] , [19] , [20] , [21] . Evidence is emerging that some miRNAs might have essential roles in haematopoiesis and leukemogenesis [22] , [23] . We reported previously that miR-196b, a miRNA located adjacent to HOXA9 , was also aberrantly overexpressed in MLL -rearranged AML, and its knockdown by antagomir abrogated MLL -fusion-mediated cell immortalization [24] . In addition, Grimes and colleagues [25] reported recently that antagomir-mediated inhibition of miR-196b function dramatically delayed MLL-AF9 -mediated leukemogenesis in vivo . Thus, miR-196b likely functions as an oncogene and appears to be required for MLL -fusion-mediated cell transformation and leukemogenesis. Surprisingly, both HOXA9 and MEIS1 are predicted targets of miR-196b, although they are co-expressed in MLL -rearranged leukaemia. As they all likely function as oncogenes, one may expect that there is some mechanism(s) leading to the loss of repression of miR-196b on HOXA9 / MEIS1 expression in leukaemia cells, but we found that this is not the case. In this study, we observed that forced expression of miR-196b significantly inhibited MLL -fusion-mediated leukemogenesis in primary mouse bone marrow transplantation (BMT), but resulted in much more aggressive leukaemic phenotypes and a faster leukemogenesis in secondary BMT recipient mice. We then showed that miR-196b could repress expression of both oncogenic (for example, HOXA9/MEIS1 ) and tumour-suppressor (for example, FAS ) target genes, indicating that miR-196b has a dual role in MLL -fusion-mediated leukemogensis. miR-196b is co-expressed with HOXA / MEIS1 in MLL leukaemia We previously showed that miR-196b was significantly overexpressed in MLL -associated AML ( Supplementary Fig. S1a ) in a bead-based miRNA profiling of 57 samples [24] , [26] , which was confirmed in our subsequent Exiqon miRNA array assay of an independent set of 85 (70 untreated and 15 relapsed; Supplementary Table S1 ) AML and 15 normal control samples ( Supplementary Fig. S1b ). We also performed Agilent Custom Gene Array assay (Agilent Technologies Inc., Santa Clara, CA, USA) of 56 untreated AML and 9 normal bone marrow (BM) samples from above samples. Through correlating miRNA and mRNA expression profiles of the 65 samples, we found that miR-196b exhibited a significantly positive correlation of expression with a group of HOXA genes and MEIS1 , and all of them were highly expressed in MLL -associated AML ( Fig. 1a ). The strong co-expression between miR-196b and HOXA genes has also been observed in acute lymphoblastic leukaemia (ALL) [27] . In contrast, other HOX genes and MEIS3 were not coexpressed with miR-196b in MLL -associated AML ( Supplementary Fig. S1c ). As the human miR-196b is located at chromosome band 7p15.2, between the loci of HOXA9 and HOXA10 ( Fig. 1a ), their co-expression suggests that they might be co-regulated. 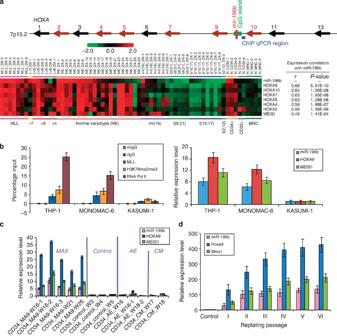Figure 1: Co-expression of miR-196b withHOXAgenes andMEIS1in human AMLs. (a) Schematic representation of the genomic organization of miR-196b andHOXAgenes, and expression correlation between miR-196b andHOXAgenes andMEIS1in 56de novoAML and 9 normal control samples. Expression data were mean centred. Red represents a high expression. N_, normal control; MNC, mononuclear cells;r, correlation coefficient. (b) Mixed lineage leukaemia (MLL) fusions bind to the upstream region of miR-196b (left panel) and promote its expression (right panel) inMLL-rearranged AML cells as detected by quantitative PCR (qPCR). (c,d) Expression of miR-196b,HOXA9andMEIS1was upregulated in human CD34+umbilical cord blood cells after retroviral transduction ofMLL-AF9(MA9) at different time points (W, week), but not in those transduced withAML1-ETO(AE) orCBFB-MYH11(CM) (c), and in mouse BM Lin−progenitor cells transduced withMLL-AF9in colony-forming/replating assays (d). The stand errors (s.e.) were based on two independent qPCR assays, and in each qPCR assay we had triplicates for each sample/reaction. Figure 1: Co-expression of miR-196b with HOXA genes and MEIS1 in human AMLs. ( a ) Schematic representation of the genomic organization of miR-196b and HOXA genes, and expression correlation between miR-196b and HOXA genes and MEIS1 in 56 de novo AML and 9 normal control samples. Expression data were mean centred. Red represents a high expression. N_, normal control; MNC, mononuclear cells; r , correlation coefficient. ( b ) Mixed lineage leukaemia (MLL) fusions bind to the upstream region of miR-196b (left panel) and promote its expression (right panel) in MLL -rearranged AML cells as detected by quantitative PCR (qPCR). ( c,d ) Expression of miR-196b, HOXA9 and MEIS1 was upregulated in human CD34 + umbilical cord blood cells after retroviral transduction of MLL-AF9 (MA9) at different time points (W, week), but not in those transduced with AML1-ETO (AE) or CBFB-MYH11 (CM) ( c ), and in mouse BM Lin − progenitor cells transduced with MLL-AF9 in colony-forming/replating assays ( d ). The stand errors (s.e.) were based on two independent qPCR assays, and in each qPCR assay we had triplicates for each sample/reaction. Full size image Evidence is emerging that MLL fusion proteins bind directly to the loci of HOXA and MEIS1 genes, and enhance their expression directly through recruiting RNA polymerase II and DOT1L-mediated methylation of histone H3 lysine 79 (H3K79) [28] , [29] , [30] , [31] . To determine whether MLL fusions also bind directly to the upstream region of miR-196b in human leukaemia cells as we had shown previously in mouse embryonic fibroblast cells [24] , we performed a chromatin immunoprecipitation assay, followed by quantitative PCR (qPCR) assay (see qPCR region location in Fig. 1a ). As expected, we observed a significant enrichment of MLL fusion proteins, methylated H3K79 and RNA polymerase II in the upstream region of miR-196b ( Fig. 1b ), which was associated with a higher expression level of the genes in MLL -rearranged leukaemia cells including THP1/t(9;11) and MONOMAC6/t(9;11), than that in non- MLL -rearranged leukaemia cells such as KASUMI-1/t(8;21) ( Fig. 1b ). Furthermore, we showed that forced expression of MLL-AF9 could significantly ( P <0.05; two-tailed t -test) increase the expression of miR-196b, HOXA9/Hoxa9 and MEIS1/Meis1 in both human umbilical cord blood CD34 + stem cells ( Fig. 1c ) and mouse haematopoietic progenitor cells ( Fig. 1d ), confirming their direct upregulation by MLL fusions. miR-196b represses expression of HOXA9 and MEIS1 Interestingly, both HOXA9 and MEIS1 are putative targets of miR-196b ( Fig. 2a ), which was confirmed by our luciferase reporter and mutagenesis assays in Hela ( Fig. 2b ) or 293T cells. Western blot analysis revealed that HOXA9 and MEIS1 protein levels were significantly reduced by forced expression of miR-196b, and increased through inhibition of miR-196b in Hela cells ( Fig. 2b ). However, due to their essential oncogenic roles [3] , [5] , [6] , [7] , [8] , [11] , [32] , it might be possible that HOXA9 and MEIS1 are not repressed by miR-196b in MLL -rearranged leukaemia. To test this hypothesis, we first sequenced 15 MLL -rearranged leukaemia patient samples along with five human normal BM control samples, but did not find any mutations or single-nucleotide polymorphisms in either the precursor of miR-196b or the genomic DNA or mRNA of the 3′ UTRs of HOXA9 and MEIS1 that would disrupt the repression. 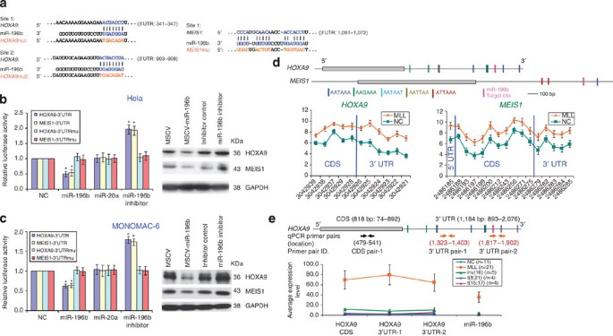Figure 2:HOXA9andMEIS1are direct targets of miR-196b. (a) Predicted target sites and relevant mutation sequences. (b,c) Luciferase reporter/mutagenesis assay (left panel) and western blotting (right panel) indicate thatHOXA9andMEIS1are repressed by miR-196b in both Hela (b) and MONOMAC6 leukaemic (c) cells. Increase in luciferase activity upon inhibition of miR-196b is due to inhibition of the endogenous expression of miR-196b. The NC (that is, negative control) for miRNA overexpression (using MSCV-miRNA) is the empty vector (that is, MSCV). miR-20a is a negative-control miRNA (for miR-196b overexpression) that consumes the same Dicer machinery in cells as miR-196b, but is predicted not to bind to the 3′ UTR of eitherHOXA9orMEIS1.The NC for miR-196b hairpin inhibitor is hairpin inhibitor negative control (that is, scrambled oligos). *P<0.05, two-tailedt-test of three independent experiments. (d) Schematic representation ofHOXA9orMEIS1mRNA, highlighted with alternative polyadenylation sites and putative miR-196b targeting sites in 3′ UTR. Grey boxes show protein-coding (CDS) regions. Average expression levels of different probes ofHOXA9orMEIS1in 15MLL-rearranged AML and 9 normal controls as detected by Affymetrix Human Exon 1.0 ST array analysis were shown. (e) Schematic illustration of three pairs of qPCR primers to analyse expression of CDS and 3′ UTR ofHOXA9. Then, qPCR analysis of CDS and 3′ UTR region ofHOXA9in 35 leukaemia and 11 normal control samples was shown. Mean±s.e. values are shown. Figure 2: HOXA9 and MEIS1 are direct targets of miR-196b. ( a ) Predicted target sites and relevant mutation sequences. ( b,c ) Luciferase reporter/mutagenesis assay (left panel) and western blotting (right panel) indicate that HOXA9 and MEIS1 are repressed by miR-196b in both Hela ( b ) and MONOMAC6 leukaemic ( c ) cells. Increase in luciferase activity upon inhibition of miR-196b is due to inhibition of the endogenous expression of miR-196b. The NC (that is, negative control) for miRNA overexpression (using MSCV-miRNA) is the empty vector (that is, MSCV). miR-20a is a negative-control miRNA (for miR-196b overexpression) that consumes the same Dicer machinery in cells as miR-196b, but is predicted not to bind to the 3′ UTR of either HOXA9 or MEIS1. The NC for miR-196b hairpin inhibitor is hairpin inhibitor negative control (that is, scrambled oligos). * P <0.05, two-tailed t -test of three independent experiments. ( d ) Schematic representation of HOXA9 or MEIS1 mRNA, highlighted with alternative polyadenylation sites and putative miR-196b targeting sites in 3′ UTR. Grey boxes show protein-coding (CDS) regions. Average expression levels of different probes of HOXA9 or MEIS1 in 15 MLL -rearranged AML and 9 normal controls as detected by Affymetrix Human Exon 1.0 ST array analysis were shown. ( e ) Schematic illustration of three pairs of qPCR primers to analyse expression of CDS and 3′ UTR of HOXA9 . Then, qPCR analysis of CDS and 3′ UTR region of HOXA9 in 35 leukaemia and 11 normal control samples was shown. Mean±s.e. values are shown. Full size image Second, it was reported that under stress (for example, oxidative stress, nutrient deprivation or DNA damage), some miRNAs may switch from a normal repressor into an activator of their targets [33] , [34] . To determine whether the potential oncogenic stress mediated by MLL fusions could cause such a switch in the regulatory mode of miR-196b, we performed luciferase reporter assays in Hela or 293T cells at 24, 48 or 96 h post transfection of MLL-AF9 , but did not observe such a switch. In a leukaemia cell line, MONOMAC6 bearing t(9;11), the repression of HOXA9 and MEIS1 by miR-196b was still present, as shown by luciferase reporter assays and western blot ( Fig. 2c ). Thus, our data suggest that under potential oncogenic stress, miR-196b still represses the expression of target genes. Finally, recent studies suggest that the loss of miRNA complementary sites through truncation of 3′ UTRs by alternative cleavage and polyadenylation might be a common mechanism of oncogene activation [35] , [36] , [37] . Indeed, we found that the 3′ UTRs of both HOXA9 and MEIS1 contain multiple putative alternative polyadenylation sites ( Fig. 2d ). This intrigued us to investigate whether there is a truncated 3′ UTR in HOXA9 and MEIS1 that prevents miR-196b-mediated repression in MLL- rearranged leukaemia. However, our Affymetrix Human Exon 1.0 ST array analysis of 15 MLL -rearranged AML and 9 normal control samples showed that there were no significant truncations of the 3′ UTR of HOXA9 or MEIS1 in MLL -rearranged AML relative to the normal controls ( Fig. 2d ). Similarly, our qPCR analysis of 21 MLL -rearranged leukaemia, 13 other leukaemia and 11 normal control samples also showed no 3′ UTR truncation of HOXA9 in MLL -rearranged leukaemia ( Fig. 2e ). miR-196b overexpression delays leukemogenesis in primary BMT As forced expression of miR-196b can significantly repress the expression of HOXA9 and MEIS1 , we further assessed its function in leukemogenesis. We co-transduced MSCV-PIG (bearing a PGK-puromycin-IRES-GFP cassette) or MSCV-PIG-miR-196b together with MSCVneo, MSCVneo- MLL-AF9 or MSCVneo- MLL-ELL into the mouse foetal liver cells (E14.5; C57BL/6) and then transplanted the cells into lethally irradiated C57BL/6 recipient mice. We found that forced expression of miR-196b significantly delayed leukemogenesis mediated by MLL-AF9 (median overall survival (OS), 62 days versus 54 days; P <0.002; log-rank test) or MLL-ELL (median OS, 179 days versus 138 days; P <0.0001; log-rank test) ( Supplementary Fig. S2 ). The above transplanted cells were unpurified and thus very heterogeneous. To validate the above results, we co-transduced MSCV-PIG or MSCV-PIG-miR-196b together with MIY (bearing YFP) or MIY- MLL-AF9 into the mouse foetal liver cells (E14.5; C57BL/6; CD45.2). Then, GFP + /YFP + cells were isolated by flow cytometry and transplanted into lethally irradiated B6.SJL (CD45.1) recipient mice. The miR-196b+ MLL-AF9 mice developed AML much slower than MLL-AF9 mice (median OS, 75 days versus 32 days; P <2.3×10 −5 ; log-rank test) ( Figures 3a and b ; Supplementary Table S2 ). 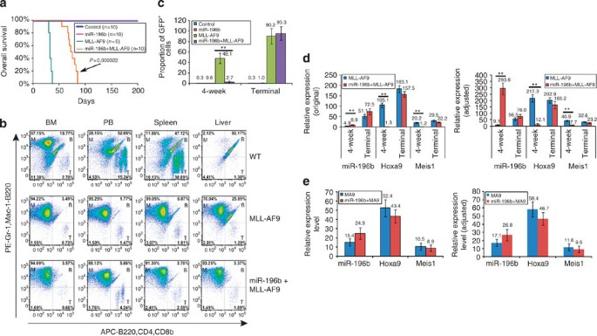Figure 3: Forced expression of miR-196b significantly delays leukemogenesis in primary transplantation. (a) Kaplan–Meier survival analysis of the mice. n, mouse number. (b) Flow cytometric analysis of bone marrow (BM), peripheral blood (PB), spleen and liver of representative mice. M, myeloid cells; B, B cells; T, T cells. (c) Engraftment degrees (that is, GFP+cell proportions) of different cohorts of transplanted mice at 4 weeks post transplantation or at the terminal stage (that is, when leukaemic mice were killed, or at 200 days post transplantation for the non-leukemic mice). (d,e) The original (left panel) and adjusted (by engraftment degree; right panel) expression levels of miR-196b,Hoxa9orMeis1in peripheral blood (PB;d) of mice at the two stages, or in BM cells (e) at the terminal stage, relative to the expression levels in PB or BM of control mice bearing retrovirally transduced empty vectors (that is, MSCV-PIG+MIY). *P<0.05; **P<0.01; two-tailedt-test. Figure 3: Forced expression of miR-196b significantly delays leukemogenesis in primary transplantation. ( a ) Kaplan–Meier survival analysis of the mice. n, mouse number. ( b ) Flow cytometric analysis of bone marrow (BM), peripheral blood (PB), spleen and liver of representative mice. M, myeloid cells; B, B cells; T, T cells. ( c ) Engraftment degrees (that is, GFP + cell proportions) of different cohorts of transplanted mice at 4 weeks post transplantation or at the terminal stage (that is, when leukaemic mice were killed, or at 200 days post transplantation for the non-leukemic mice). ( d,e ) The original (left panel) and adjusted (by engraftment degree; right panel) expression levels of miR-196b, Hoxa9 or Meis1 in peripheral blood (PB; d ) of mice at the two stages, or in BM cells ( e ) at the terminal stage, relative to the expression levels in PB or BM of control mice bearing retrovirally transduced empty vectors (that is, MSCV-PIG+MIY). * P <0.05; ** P <0.01; two-tailed t -test. Full size image To reveal the mechanism underlying the longer latency caused by miR-196b, we analysed engraftment history of the mice. Strikingly, we found that the proportion of GFP + cells in peripheral blood (PB) of miR-196b+ MLL-AF9 mice 4 weeks post transplantation is 2.7% on average, dramatically ( ∼ 18-fold; P <0.01, two-tailed t -test) lower than that (48.1%) of MLL-AF9 mice ( Fig. 3c ), indicating that forced expression of miR-196b significantly inhibited engraftment. After adjusting for the level of engraftment, we found that the expression level of miR-196b in PB of miR-196b+ MLL-AF9 mice is dramatically (>32-fold; P <0.01, two-tailed t -test) higher at 4 weeks post transplantation whereas it is only slightly (1.4-fold) higher at the terminal stage (that is, at the time to be killed with fully developed leukaemia) than that of MLL-AF9 mice ( Fig. 3d ). The relative decrease of miR-196b expression in miR-196b+ MLL-AF9 mice from the 4-week stage to the terminal stage is likely due to the gradual transcriptional silencing of retroviral vectors (for example, MSCV) in haematopoietic stem cells as reported previously [38] , [39] . Accordingly, the mRNA expression level of Hoxa9 and Meis1 in PB of miR-196b+ MLL-AF9 mice was significantly (20–100-fold; P <0.01, two-tailed t -test) lower in the beginning but only slightly lower at the terminal stage than that of MLL-AF9 mice ( Fig. 3d ). The relative RNA expression levels of miR-196b, Hoxa9 and Meis1 in BM cells at the terminal stage showed the same pattern as those in PB ( Fig. 3e ). Interestingly, the higher level of miR-196b expression in the initial stage is largely associated with the longer latency. Therefore, the dramatically higher expression level of miR-196b in the initial stage dramatically inhibited expression of Hoxa9 and Meis1 , which leads to a much lower engraftment and thereby a significantly longer latency. The miR-196b+ MLL-AF9 -induced leukaemia is more aggressive Based on the above data, one might expect that miR-196b is a tumour-suppressor gene in leukemogenesis, which, however, is contradictory to the previous findings that miR-196b functions as an oncogene and is required for the MLL -fusion-mediated cell transformation and leukemogenesis [24] , [25] . Indeed, consistent with the oncogenic role of miR-196b, we found that miR-196b+ MLL-AF9 leukaemia cells had a higher proportion of immature blast cells than MLL-AF9 leukaemic cells in both PB and BM, and leukaemia cell infiltration and disruption of organ architecture in liver and spleen seemed to be more aggressive in miR-196b+ MLL-AF9 mice than in MLL-AF9 mice ( Fig. 4a ). Colony-forming assay analysis showed that leukaemic BM cells from miR-196b+ MLL-AF9 mice formed 6-fold more colonies than those from MLL-AF9 mice ( Fig. 4b ), implying that the proportion of leukaemia stem/initiating cells in BM is much higher in miR-196b+ MLL-AF9 than that in MLL-AF9 mice. 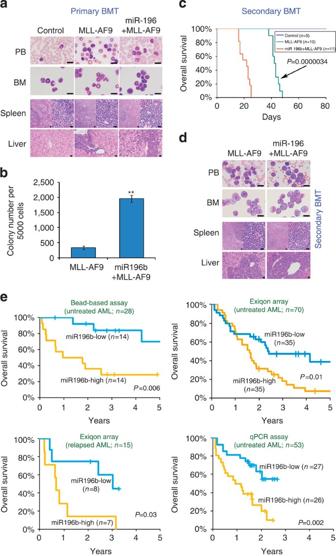Figure 4: Overexpression of miR-196b is associated with aggressive leukaemia in mice and poor prognosis in acute myeloid leukaemia (AML) patients. (a) Comparison ofMLL-AF9and miR-196b+MLL-AF9primary leukaemic cells and tissues. (b) Colony-forming assay of primary leukaemic bone marrow (BM) cells. Plated 5,000 cells per dish and cultured for 7 days before count. BM cells isolated from three leukaemic mice in each group were used for the assay. **P<0.01, two-tailedt-test. (c) Kaplan–Meier survival analysis of the secondary transplantation mice. Mouse number. (d) Comparison ofMLL-AF9and miR-196b+MLL-AF9secondary leukaemic cells and tissues. Peripheral blood (PB) smear and BM cell cytospinviaWright–Giemsa staining, and spleen and liver tissuesviahaematoxylin and eosin (H&E) staining of paraffin sections (resolution is indicated on the images) are shown. (e) Patients with increased expression of miR-196b exhibited significantly (P<0.05; log-rank test) shorter overall survival (OS) than those with decreased expression in different patient sets. Each AML patient set was dichotomized at the median value of miR-196b expression, and Kaplan–Meier curves were generated to depict outcomes.∣, censored. The length of bars shown in (a) and (d) represents 10 μm (for PB and BM) or 50 μm (for spleen and liver tissues). BMT, bone marrow transplantation. Figure 4: Overexpression of miR-196b is associated with aggressive leukaemia in mice and poor prognosis in acute myeloid leukaemia (AML) patients. ( a ) Comparison of MLL-AF9 and miR-196b+ MLL-AF9 primary leukaemic cells and tissues. ( b ) Colony-forming assay of primary leukaemic bone marrow (BM) cells. Plated 5,000 cells per dish and cultured for 7 days before count. BM cells isolated from three leukaemic mice in each group were used for the assay. ** P <0.01, two-tailed t -test. ( c ) Kaplan–Meier survival analysis of the secondary transplantation mice. Mouse number. ( d ) Comparison of MLL-AF9 and miR-196b+ MLL-AF9 secondary leukaemic cells and tissues. Peripheral blood (PB) smear and BM cell cytospin via Wright–Giemsa staining, and spleen and liver tissues via haematoxylin and eosin (H&E) staining of paraffin sections (resolution is indicated on the images) are shown. ( e ) Patients with increased expression of miR-196b exhibited significantly ( P <0.05; log-rank test) shorter overall survival (OS) than those with decreased expression in different patient sets. Each AML patient set was dichotomized at the median value of miR-196b expression, and Kaplan–Meier curves were generated to depict outcomes. ∣ , censored. The length of bars shown in ( a ) and ( d ) represents 10 μm (for PB and BM) or 50 μm (for spleen and liver tissues). BMT, bone marrow transplantation. Full size image We then transplanted BM cells isolated from two each of the control, miR-196b+ MLL - AF9 , and MLL-AF9 mice, respectively, into sublethally irradiated secondary recipient mice (B6.SJL). Consistent with their more aggressive properties already shown ( Fig. 4a,b ), miR-196b+ MLL-AF9 leukaemic cells developed AML in secondary recipient mice significantly faster than MLL-AF9 leukaemic cells (median OS, 19 days versus 42 days; P <0.000004, log-rank test; Fig. 4c ). Both groups had comparable immature cells in PB and BM, but the disruption of structure in spleen and liver seemed to be more severe in miR-196b+ MLL-AF9 mice than that in MLL-AF9 mice ( Fig. 4d ). These findings suggest that miR-196b does have an oncogenic role in MLL -rearranged leukaemia. Overexpression of miR-196b is associated with adverse survival We then assessed the prognostic impact of miR-196b expression in AML patients. Through Cox regression analyses of the AML patients included in the bead-based miRNA profiling [26] ( n =28), Exiqon miRNA array (de novo AML, n =70; relapsed AML, n =15; Supplementary Fig. S1 ) and qPCR assay [40] ( n =53), we found that increased expression of miR-196b was significantly ( P <0.05, Cox regression) associated with shorter OS of AML patients ( Supplementary Table S3 ). Kaplan–Meier curve analyses showed that the patients with a higher level of miR-196b expression exhibited a significantly ( P <0.05, log-rank test) shorter survival than those with a lower level in all patient sets ( Fig. 4e ). Through multivariable testing in the largest patient set ( n =70), we found that miR-196b expression signature was an independent predictor of outcome in AML after adjusting for other variables ( Supplementary Table S4 ). miR-196b also targets tumour-suppressor genes such as Fas The above results suggest that miR-196b must also target some critical tumour-suppressor genes, which contributes to the more aggressive leukaemic phenotypes. To identify such targets, we conducted Affymetrix gene arrays of leukaemic BM samples from 24 mice including 9 primary (including 3 each of negative control, MLL-AF9 and miR-196b+ MLL-AF9 ) and 15 secondary (including 3 negative control, 6 MLL-AF9 and 6 miR-196b+ MLL-AF9 ) recipient mice. Through significance analysis of microarrays [41] , we identified 897 genes that were significantly downregulated ( q <0.05) in all the 18 leukaemia samples relative to the 6 negative controls, and 116 were expressed at a further significantly ( q <0.05) lower level in miR-196b+ MLL-AF9 than in MLL-AF9 leukaemic cells. Of the 116 genes, 41 genes are predicted as putative targets of miR-196b ( Fig. 5a ). We then performed Affymetrix exon array assay of 15 human MLL -rearranged samples and 9 human normal (including 3 each of CD34 + , CD33 + and mononuclear cells) BM samples, and found that 17 out of the 41 candidates were significantly ( q <0.05; significance analysis of microarrays) downregulated in MLL -rearranged leukaemia relative to normal CD33+ and mononuclear cell samples ( Fig. 5b ). Furthermore, in a set of 485 AML patients (namely Netherlands-AML-Set; Supplementary Table S1 ) [42] , we found that among the above 17 candidate targets, only the downregulation of FAS was significantly ( P <0.05; Cox regression) associated with shorter OS and event-free survival ( Supplementary Tables S5 and S6 ; Fig. 5c ), in accordance with the association between upregulation of miR-196b and poor survival ( Fig. 4e ; Supplementary Tables S3 and S4 ). The association of downregulation of FAS with poor outcome was also observed in previous small-scale (patient number<40) studies [43] , [44] , [45] , [46] . In multivariable testing, the downregulation of FAS expression was shown as an independent predictor of poor survival after adjusting for other variables ( Supplementary Table S7 ). Meanwhile, F AS is a putative target of miR-196b as predicted by all the four programmes ( Fig. 5 ). Therefore, we chose FAS as an important tumour-suppressor candidate target of miR-196b for further studies. 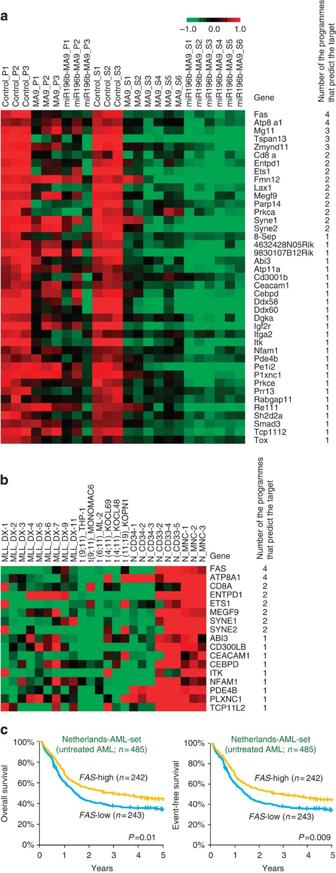Figure 5: Candidate target genes of miR-196b. (a) Gene expression profiles of 41 predicted target genes of miR-196b in BM cells of primary and secondary transplantation mice as detected by Affymetrix mouse gene arrays. Expression data were mean centred and the relative value for each sample is represented by a colour, with red representing a high expression and green representing a low expression (scale shown in the upper left).MA9,MLL-AF9; _P, primary transplantation recipient mouse; _S, secondary transplantation recipient mouse. (b) Seventeen out of the above 41 candidate target genes of miR-196b were also significantly (q<0.05; FDR<0.01; significance analysis of microarrays (SAM)41) downregulated in humanMLL-rearranged leukaemia samples relative to human normal CD33+myeloid and mononuclear cell (MNC) samples. Normal CD34+stem/progenitor cell samples were not included in the SAM analysis. Expression data were mean centred and the relative value for each sample is represented by a colour, with red representing a high expression and green representing a low expression (scale shown in the upper left). (c) Patients with decreased expression ofFASexhibited significantly (P<0.05; log-rank test) shorter OS and event-free survival (EFS) than those with increased expression. Each acute myeloid leukaemia (AML) patient set was dichotomized at the median value ofFASexpression, and Kaplan–Meier curves were generated to depict outcomes. |, censored. Figure 5: Candidate target genes of miR-196b. ( a ) Gene expression profiles of 41 predicted target genes of miR-196b in BM cells of primary and secondary transplantation mice as detected by Affymetrix mouse gene arrays. Expression data were mean centred and the relative value for each sample is represented by a colour, with red representing a high expression and green representing a low expression (scale shown in the upper left). MA9 , MLL-AF9 ; _P, primary transplantation recipient mouse; _S, secondary transplantation recipient mouse. ( b ) Seventeen out of the above 41 candidate target genes of miR-196b were also significantly ( q <0.05; FDR<0.01; significance analysis of microarrays (SAM) [41] ) downregulated in human MLL -rearranged leukaemia samples relative to human normal CD33 + myeloid and mononuclear cell (MNC) samples. Normal CD34 + stem/progenitor cell samples were not included in the SAM analysis. Expression data were mean centred and the relative value for each sample is represented by a colour, with red representing a high expression and green representing a low expression (scale shown in the upper left). ( c ) Patients with decreased expression of FAS exhibited significantly ( P <0.05; log-rank test) shorter OS and event-free survival (EFS) than those with increased expression. Each acute myeloid leukaemia (AML) patient set was dichotomized at the median value of FAS expression, and Kaplan–Meier curves were generated to depict outcomes. |, censored. Full size image The downregulation of FAS in human MLL -rearranged leukaemic cells was further confirmed by qPCR ( Fig. 6a ). In PB of primary BMT mice, Fas expression was significantly ( P <0.05; two-tailed t -test) downregulated in both MLL-AF9 and, particularly, miR-196b+ MLL-AF9 (especially at the initial stage) than in normal control samples ( Fig. 6b ). Through luciferase reporter/mutagenesis assays, we showed that FAS is a direct target of miR-196b ( Fig. 6c ). Western blot assay showed that endogenous expression of Fas was significantly repressed by miR-196b in primary and secondary leukaemic BM cells ( Fig. 6d ). 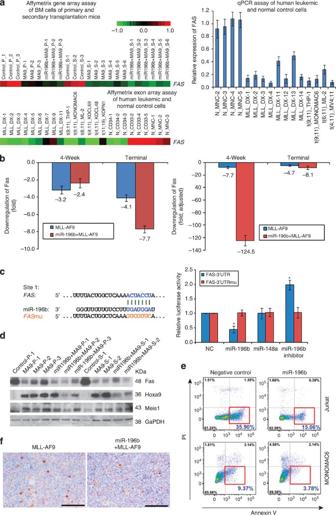Figure 6:Fasis a direct target of miR-196b. (a) Expression profiles ofFAS/Fasby Affymetrix gene array and affymetrix exon array assays (left panel); Expression ofFasby quantitative PCR (qPCR) assay (right panel). (b) The original (left panel) and adjusted (by engraftment degree; right panel) expression levels ofFasin PB of primary BMT mice at the two stages, relative to the expression levels in PB of control mice bearing retrovirally transduced empty vectors (that is, MSCV-PIG+MIY). (c) Wild-type and mutated target site of miR-196b in 3′ UTR ofFAS(left panel), and luciferase reporter and mutagenesis assays (right panel). NC, negative control. miR-148 is a control miRNA that is predicted not to targetFAS. *P<0.05, two-tailedt-test of three independent experiments. (d) Western blotting assay of Fas, Hoxa and Meis1 in bone marrow (BM) cells of primary (P-) and secondary (S-) transplantation mice. (e) Flow cytometry analysis of anti-Fas antibody-induced apoptosis in Jurkat and MONOMAC6 cells with or without ectopic expression of miR-196b. (f) Immunohistochemical staining of paraffin-embedded secondary transplantation spleen tissues with cleaved caspase-3 antibody. The apoptotic cells are shown in brown; apoptotic cells per field in miR-196b+MLL-AF9 tissue is 6, much fewer than that (19) in MLL-AF9 tissue. The length of the bars represents 50 μm. Figure 6: Fas is a direct target of miR-196b. ( a ) Expression profiles of FAS/Fas by Affymetrix gene array and affymetrix exon array assays (left panel); Expression of Fas by quantitative PCR (qPCR) assay (right panel). ( b ) The original (left panel) and adjusted (by engraftment degree; right panel) expression levels of Fas in PB of primary BMT mice at the two stages, relative to the expression levels in PB of control mice bearing retrovirally transduced empty vectors (that is, MSCV-PIG+MIY). ( c ) Wild-type and mutated target site of miR-196b in 3′ UTR of FAS (left panel), and luciferase reporter and mutagenesis assays (right panel). NC, negative control. miR-148 is a control miRNA that is predicted not to target FAS . * P <0.05, two-tailed t -test of three independent experiments. ( d ) Western blotting assay of Fas, Hoxa and Meis1 in bone marrow (BM) cells of primary (P-) and secondary (S-) transplantation mice. ( e ) Flow cytometry analysis of anti-Fas antibody-induced apoptosis in Jurkat and MONOMAC6 cells with or without ectopic expression of miR-196b. ( f ) Immunohistochemical staining of paraffin-embedded secondary transplantation spleen tissues with cleaved caspase-3 antibody. The apoptotic cells are shown in brown; apoptotic cells per field in miR-196b+MLL-AF9 tissue is 6, much fewer than that (19) in MLL-AF9 tissue. The length of the bars represents 50 μm. Full size image Consistent with the previous findings that the downregulation of FAS is associated with decreased apoptosis [47] , we also found that ectopic expression of miR-196b significantly inhibited FAS antibody-induced apoptosis in both Jurkat (35.9% versus 15.06%) and MONOMAC6 (9.37% versus 3.78%) cells ( Fig. 6e ). Accordingly, immunohistochemical staining of spleen tissues with cleaved caspase-3 antibody showed that miR-196b+ MLL-AF9 cells had a much lower frequency of apoptosis than MLL-AF9 cells ( Fig. 6f ). These data indicate that forced expression of miR-196b induced severe leukaemia in primary MLL -rearranged leukaemic cells and shorter latency in secondary leukaemia likely through targeting Fas . Fas expression suppresses MLL-AF9 -mediated leukemogenesis To validate the role of Fas in MLL -rearranged leukaemia, we forced the expression of FAS -coding region (that is, CDS, does not contain 3′ UTR) in both miR-196b+ MLL-AF9 and MLL-AF9 primary leukaemic BM cells. We found that Fas overexpression significantly delayed the development of leukaemia in secondary transplantation (median OS, 54 days versus 37 days, P <0.05, log-rank test, from miR-196b+ MLL-AF9 donor cells; median OS, 83 days versus 62 days, P <0.05, log-rank test, from MLL-AF9 donor cells) ( Fig. 7a ). There were fewer immature cells and more apoptotic cells in PB, BM, spleen and liver of FAS -overexpressing mice ( Figs 7b,c ). The structure of spleen and liver was better maintained ( Fig. 7b ), and size of spleen and liver was significantly smaller ( P <0.05; two-tailed t -test) in FAS -overexpressing mice compared with that of control mice ( Supplementary Table S8 ). These results suggest that FAS expression suppresses MLL -rearranged leukaemia likely through induction of apoptosis, indicating that miR-196b repression of FAS is important in the development of MLL-fusion-mediated leukemogenesis. 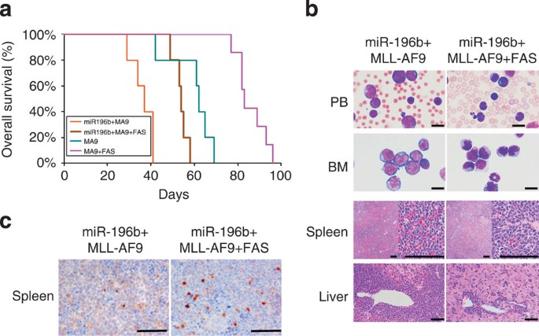Figure 7: Forced expression ofFASinhibits leukemogenesis in secondary transplantation. (a) Kaplan–Meier survival analysis of mice. MA9, MLL-AF9. (b) Comparison of miR-196b+MLL-AF9with or withoutFAS-overexpressing secondary leukaemic cells and tissues. (c) Immunohistochemical staining of paraffin-embedded secondary transplantation spleen tissues with cleaved caspase-3 antibody. The apoptotic cells are shown in brown; apoptotic cells per field in miR-196b+MLL-AF9 tissue is 8, much fewer than that (30) in miR-196b+MLL-AF9+FAS tissue. The length of bars shown inFigure 7b,crepresents 10 μm (for peripheral blood (PB) and bone marrow (BM)) or 50 μm (for spleen and liver tissues). Figure 7: Forced expression of FAS inhibits leukemogenesis in secondary transplantation. ( a ) Kaplan–Meier survival analysis of mice. MA9, MLL-AF9. ( b ) Comparison of miR-196b+ MLL-AF9 with or without FAS -overexpressing secondary leukaemic cells and tissues. ( c ) Immunohistochemical staining of paraffin-embedded secondary transplantation spleen tissues with cleaved caspase-3 antibody. The apoptotic cells are shown in brown; apoptotic cells per field in miR-196b+MLL-AF9 tissue is 8, much fewer than that (30) in miR-196b+MLL-AF9+FAS tissue. The length of bars shown in Figure 7b,c represents 10 μm (for peripheral blood (PB) and bone marrow (BM)) or 50 μm (for spleen and liver tissues). Full size image miR-196b regulates Hoxa9 / Meis1 and Fas in haematopoiesis To analyse expression correlation between miR-196b and target genes in normal haematopoiesis, we isolated murine long-term haematopoietic stem cells, short-term HSCs (ST-HSCs), committed progenitors (CPs), lineage negative (Lin − ) progenitor cells, myeloid (Gr-1 + /Mac-1 + ) and lymphoid (B220 + ) cells. 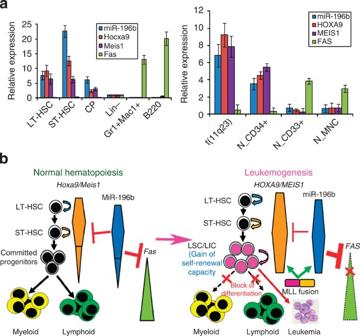Figure 8: Regulation ofHoxa9/Meis1andFasexpression by miR-196b in haematopoiesis and leukemogenesis. (a) Relative expression levels of miR-196b,Hoxa9,Meis1andFasin normal haematopoietic cells (left panel) and inMLL-rearranged leukaemic cells (right panel). In mouse normal haematopoietic cells, their expression levels in long-term HSC (LT-HSC; Lin−Sca1+c-Kit+Flk2−, LSKF−), short-term HSC (ST-HSC; Lin−Sca1+c-Kit+Flk2+, LSKF+), committed progenitor (CP; Lin−Sca1−c-Kit+), Gr-1+/Mac-1+myeloid and B220+lymphoid cells, were normalized by the levels in lineage negative (Lin−) cells. In humanMLL-rearranged leukaemic cells, their expression levels in normal CD34+(N_CD34+) haematopoietic stem/progenitor cells, normal CD33+(N_CD33+) myeloid cells and mononuclear cells (MNC) were normalized by the mean expression values of all the normal control samples. (b) Model of miR-196b-mediated gene regulations in normal haematopoiesis (left panel) and humanMLL-associated leukemogensis (right panel). In haematopoiesis, miR-196b contributes to the fine tuning of expression abundance ofHoxa9andMeis1while repressing expression ofFasduring haematopoiesis, particularly in the period of ST-HSC and committed progenitor cells; once expression of miR-196b is downregulated, expression ofFasis upregulated, which in turns promotes differentiation. In leukemogenesis, MLL fusions aberrantly upregulate expression ofHOXA9,MEIS1and miR-196b, particularly in committed progenitor cells60. Although expression ofHOXA9andMEIS1is still partially repressed by miR-196b, the residual abundance of their transcripts is adequate for cell transformation; on the other hand, expression ofFasand other tumour-suppressor target genes that are important for cell differentiation and/or apoptosis has been thoroughly inhibited by miR-196b due to the extra high level of miR-196b expression. As a result, the committed progenitor cells carryingMLL-fusion lose their capacity to differentiate while regaining self-renewal capacity, and thereby are transformed into leukaemia stem/initiating cells (LSC or LIC) and eventually cause leukaemia. As shown in Figure 8a (left panel), relative to the expression level in Lin − cells, Hoxa9 and Meis1 are highly expressed in LT- and ST-HSCs, and then gradually are downregulated in CPs, resulting in almost no expression in more mature myeloid (Gr-1 + /Mac-1 + ) and lymphoid (B220 + ) cells. MiR-196b exhibited a similar expression pattern to Hoxa9 and Meis1 , but the degree of upregulation of miR-196b in ST-HSCs and CPs, relative to Lin − cells, is much greater than that of Hoxa9 or Meis1 . Fas is expressed at a very low level in HSCs and CPs and then gradually is upregulated during haematopoiesis, and reaches a high level in myeloid and lymphoid cells. Figure 8: Regulation of Hoxa9 / Meis1 and Fas expression by miR-196b in haematopoiesis and leukemogenesis. ( a ) Relative expression levels of miR-196b, Hoxa9 , Meis1 and Fas in normal haematopoietic cells (left panel) and in MLL -rearranged leukaemic cells (right panel). In mouse normal haematopoietic cells, their expression levels in long-term HSC (LT-HSC; Lin − Sca1 + c-Kit + Flk2 − , LSKF − ), short-term HSC (ST-HSC; Lin − Sca1 + c-Kit + Flk2 + , LSKF + ), committed progenitor (CP; Lin − Sca1 − c-Kit + ), Gr-1 + /Mac-1 + myeloid and B220 + lymphoid cells, were normalized by the levels in lineage negative (Lin − ) cells. In human MLL -rearranged leukaemic cells, their expression levels in normal CD34 + (N_CD34 + ) haematopoietic stem/progenitor cells, normal CD33 + (N_CD33 + ) myeloid cells and mononuclear cells (MNC) were normalized by the mean expression values of all the normal control samples. ( b ) Model of miR-196b-mediated gene regulations in normal haematopoiesis (left panel) and human MLL -associated leukemogensis (right panel). In haematopoiesis, miR-196b contributes to the fine tuning of expression abundance of Hoxa9 and Meis1 while repressing expression of Fas during haematopoiesis, particularly in the period of ST-HSC and committed progenitor cells; once expression of miR-196b is downregulated, expression of Fas is upregulated, which in turns promotes differentiation. In leukemogenesis, MLL fusions aberrantly upregulate expression of HOXA9 , MEIS1 and miR-196b, particularly in committed progenitor cells [60] . Although expression of HOXA9 and MEIS1 is still partially repressed by miR-196b, the residual abundance of their transcripts is adequate for cell transformation; on the other hand, expression of Fas and other tumour-suppressor target genes that are important for cell differentiation and/or apoptosis has been thoroughly inhibited by miR-196b due to the extra high level of miR-196b expression. As a result, the committed progenitor cells carrying MLL -fusion lose their capacity to differentiate while regaining self-renewal capacity, and thereby are transformed into leukaemia stem/initiating cells (LSC or LIC) and eventually cause leukaemia. Full size image According to our present concepts or assumptions [18] , [19] , [22] , [23] , [48] , an oncogenic miRNA would selectively repress expression of its tumour-suppressor target genes in tumourigenesis, but not affect expression of oncogenic potential target genes although they also have the seed sequences for the miRNA to bind; similarly, a tumour-suppressor miRNA would selectively target oncogenes but not tumour suppressors in normal development or cell differentiation. This is the logic commonly followed by most of the investigators when they are trying to identify candidate target genes of a given miRNA. However, given the fact that a single miRNA has tens or hundreds of putative target genes [49] , usually including both oncogenes and tumour suppressors, it might not be practicable for a given oncogenic or tumour-suppressor miRNA to selectively repress the expression of only the targets with opposite functions than the miRNA. By providing compelling evidence, here, we show that a poor-prognosis-related miRNA (that is, miR-196b) could repress the expression of both oncogenic (for example, HOXA9/MEIS1 ) and tumour-suppressor (for example, FAS ) target genes simultaneously, and its repression of the critical tumour-suppressor target(s) likely has a predominant role in MLL-fusion-mediated leukemogenesis and contributes to the unfavourable prognosis of MLL -rearranged leukaemia. Notably, miR-196b is co-expressed with HOXA9/MEIS1 in MLL -rearranged leukaemia ( Fig. 1 ), suggesting that miRNAs may also target co-expressed (that is, transcriptionally positively correlated) genes. In an analysis of over 10 individual human and mouse sample sets, we found that transcriptionally positively correlated ( P <0.05; Pearson correlation) miRNA-putative target pairs are as frequent as, or even more frequent than, inversely (that is, negatively) correlated pairs (He C et al ., unpublished data), which is consistent with a previous study [50] , indicating that co-expression between miRNAs and putative targets is very common. As aforementioned, we thought in the beginning that miRNAs might not negatively regulate expression of their co-expressed target genes, particularly if they have similar functions. However, although some mechanisms such as sequence mutations or single-nucleotide polymorphisms [51] , miRNA regulatory mode switch [33] , [34] and 3′ UTR truncation [35] , [36] , [37] had been suggested to circumvent negative regulation of target genes by a given miRNA, none of them appears applicable in MLL -rearranged leukaemia to enable HOXA9/MEIS1 to escape from miR-196b-mediated repression ( Fig. 2 ). In fact, except for the few examples [33] , [34] , [35] , [36] , [37] , the loss of miRNA-mediated negative regulation through these mechanisms seems rare. Thus, the negative regulation of expression of the co-expressed target genes that have similar function to the miRNA may be common. The ability of a single miRNA (or a group of miRNAs) to target both oncogenes and tumour suppressors simultaneously, or sequentially, might be important for normal development and cell differentiation. Indeed, the potential regulation of many 3′ Hox (that is, Hox 1–9) genes by miR-196 [52] , [53] might be a highly evolutionarily conserved mechanism. In embryonic development, miR-196b may help to repress more anterior Hox programmes, and thereby reinforce the hierarchy of 5′ Hox function [54] . In normal haematopoiesis, miR-196b likely helps to fine-tune the expression of Hox genes and Meis1 in HSCs and to remove their residual transcripts in CPs to allow further differentiation of the cells; when miR-196b is downregulated, Fas becomes upregulated to maintain homoeostasis of the cells (see a model in Fig. 8b ; left panel). In human MLL -rearranged leukaemia, despite partial repression by miR-196b, HOXA9 and MEIS1 expression levels were still high enough to induce and maintain leukaemia ( Figs 1 , 2 , 3 , 6d , and right panel of Fig. 8a ), and therefore repression of Hoxa9 and Meis1 by miR-196b is not beneficial but is allowable; in contrast, repression of tumour-suppressor targets (for example, Fas ; Figs 6 , 7 and right panel of Fig. 8a ) seems required for MLL -fusion-mediated cell transformation and leukemoegensis, and thus knockdown of miR-196b expression could significantly inhibit the cell transformation and leukemogensis [24] , [25] . As a result, the oncogenic role of miR-196b overwhelms its tumour-suppressor role in MLL -rearranged leukaemia, and the higher level of its expression is associated with the more aggressive leukaemic phenotypes and the worse prognosis ( Fig. 4 ). However, in some other cases, the repression of oncogenic targets by miR-196b is more critical than its repression of tumour-suppressor targets, and as a result, the loss (or downregulation) of miR-196b expression leads to the promotion of tumourigenesis, such as in ALL [55] , [56] and breast cancer [57] . Taken together, we reported here a previously unappreciated miRNA-mediated regulatory model in which a single miRNA could repress expression of both oncogenic and tumour-suppressor target genes, though the repression of one group of targets has a more dominant role than repression of the other group in determining cell fate in normal differentiation/development or tumourigenesis. This regulatory model is likely very common, given the fact that most of individual miRNAs have both oncogenic and tumour-suppressor target genes, and it is not possible for an entire group of targets to circumvent the negative regulation of a miRNA completely. In the haematopoietic system, the dynamic change of the miR-196b-mediated gene regulation in an evolutionarily conserved spatial and temporal mode is essential for normal haematopoiesis ( Fig. 8b , left panel). However, aberrant upregulation of both miR-196b and its oncogenic targets (for example, HOXA9 and MEIS1 ) by MLL fusions results in the persistent repression of expression of its tumour-suppressor targets (for example, FAS ), along with the residual high level of HOXA9/MEIS1 , and thereby inhibits differentiation, disrupts cell homoeostasis and promotes cell proliferation via inhibiting apoptosis, and eventually results in cell transformation and leukemogenesis (see a model in Fig. 8b , right panel). It is well recognized that a single gene may function as an oncogene in some types of tissues but as a tumour suppressor in other types through a context-dependent manner (for example, Refs. 58 , 59 ). Now, our data suggest that a single miRNA may target two groups of genes with distinct functions, simultaneously, or sequentially, in the same tissue/cell context, and the miRNA-mediated regulation of a dynamic balance between the two groups of target genes is essential for the normal development and cell differentiation; disruption of such a balance by other oncogenic events (for example, chromosomal translocation) may lead to tumourigenesis. Thus, we probably should update our present concepts about miRNA regulation in normal development/cell differentiation and in tumourigenesis, as well as refining our definitions of oncogenic miRNAs or tumour-suppressor miRNAs. In addition, our data also calls for cautions if we plan to target a miRNA for cancer therapy in the future. When we plan to knock down the expression of a pro-tumour miRNA by antagomiR or restore expression of an anti-tumour miRNA by mimic oligos for clinical application, we should assess the corresponding potential expression changes of some co-expressed critical targets that exhibit similar function as the miRNA (for example, knocking down miR-196b expression in MLL -rearranged leukaemia may lead to further upregulation of HOXA9/MEIS1 ). Thus, the effect(s) of expression changes of those targets should be evaluated before the clinical application is pursued. Leukaemic patient and cell line samples All of the AML patient samples were obtained at the time of diagnosis or relapse and with informed consent at the University of Chicago Hospital (UCH) or other collaborative hospitals, and were approved by the institutional review board of the institutes/hospitals. All patients were treated according to the protocols of the corresponding institutes/hospitals. The clinical and molecular characteristics of these AML patients are shown in Supplementary Table S1 . The samples were stored in liquid nitrogen until used. Blasts and mononuclear cells were purified by use of NycoPrep 1.077A (Axis-Shield, Oslo, Norway). All cell lines were maintained in the lab. RNA extraction and quantitative RT–PCR Total RNA was extracted with the miRNeasy extraction kit (Qiagen, Valencia, CA, USA) and was used as a template to synthesize complementary DNA for quantitative RT–PCR (qPCR) analysis in a 7900HT real-time PCR system (Applied Biosystems, Foster City, CA, USA). TaqMan qPCR assay was performed to validate the differential expression patterns of miRNAs using kits from Applied Biosystems. qPCR with SYBR Green dye (Qiagen) was used to determine expression of mRNA genes. U6 RNA (for human) or snoRNA202 (for mouse) and GAPDH or PGK1 were used as endogenous controls for qPCR of miRNA and mRNA, respectively. Each sample was run in triplicate. qPCR primers are available upon request. miRNA and mRNA expression profiling assays The miRNA expression profiling assays of the 57 human (54 AML and 3 normal control) sample set and the 100 human (85 AML and 15 normal control) samples were conducted by use of a bead-based method [25] , [28] and Exiqon miRCURY LNA arrays (v10.0; covering 757 human miRNAs; Exiqon, Woburn, MA, USA), respectively. The mRNA microarrays of the 65 human (56 AML and 9 normal control) sample set, the 24 human (15 MLL -rearranged AML and 9 normal control) sample set, the 24 mouse (9 primary and 15 secondary BMT) sample set and Netherlands-AML-Set ( n =485) [42] were conducted by use of Agilent's custom-design microarrays (Agilent Technologies Inc.), Affymetrix GeneChip Human Exon 1.0 ST arrays, Affymetrix GeneChip Mouse Gene 1.0 ST arrays and Affymetrix U133 Plus2.0 arrays (Affymetirx, Santa Clara, CA, USA), respectively. DNA extraction, amplification and sequencing Genomic DNA was extracted using DNeasy Blood & Tissue Kit (Qiagen) according to the manufacturer's instructions. Primers that cover the precursor region of miR-196b were used to amplify the genomic DNA. PCR products were purified and sequenced directly. For 3′ UTR of HOXA9 and MEIS1 sequencing, RNA was reverse transcripted and amplified with One-Step RT–PCR Kit (Qiagen). PCR product was purified and sequenced. Primary BMT assays For primary BMT assays shown in Supplementary Figure S2a , normal foetal liver cells (E14.5) of C57BL/6 (CD45.2) mice were retrovirally transduced with MSCV-PIG + MSCVneo (as control), MSCV-PIG-miR-196b + MSCVneo (that is, miR-196b), MSCV-PIG + MSCVneo- MLL-AF9 (that is, MLL-AF9 ), MSCV-PIG + MSCVneo- MLL-ELL (that is, MLL-ELL ), MSCV-PIG-miR-196b + MSCVneo- MLL-AF9 (that is, miR-196b+ MLL-AF9 ) and MSCV-PIG-miR-196b + MSCVneo- MLL-ELL (that is, miR-196b+ MLL-ELL ), respectively, through two rounds of spinoculation [26] . Then, retrovirally transduced donor cells were injected by tail vein into lethally irradiated (960 rad) 8- to 10-week-old C57BL/6 (CD45.2) recipient mice with 1.0 million cells per recipient mouse. For primary BMT assays shown in Figure 3a , normal foetal liver cells (E14.5) of C57BL/6 (CD45.2) mice were retrovirally transduced with MSCV-PIG + MIY (as control), MSCV-PIG-miR-196b+MIY (that is, miR-196b), MSCV-PIG+MIY- MLL-AF9 (that is, MLL-AF9 ) and MSCV-PIG-miR-196b+MIY- MLL-AF9 (that is, miR-196b+ MLL-AF9 ), respectively, through two rounds of spinoculation [26] . GFP + /YFP + cells were further selected from the retrovirally transduced donor cells by flow cytometry, and then transplanted into lethally irradiated (960 rads) 8- to 10-week-old B6.SJL (CD45.1) recipient mice via tail vein injection, with 1×10 5 GFP + /YFP + cells plus a radioprotective dose of whole BM cells (1×10 6 ; freshly harvested from a B6.SJL mouse) per recipient mouse. Secondary BMT assays For secondary BMT assays shown in Figure 4c , leukaemic or normal control BM cells isolated from the primary recipient mice were further transplanted into sublethally irradiated (480 rads) 8- to 10-week-old B6.SJL (CD45.1) secondary recipient mice via tail vein injection, with 5×10 5 donor cells plus a radioprotective dose of whole BM cells (1x10 6 ; freshly harvested from a B6.SJL mouse) per secondary recipient mouse. For secondary BMT assays shown in Figure 7a , leukaemic BM cells isolated from the miR-196b+ MLL-AF9 or MLL-AF9 primary recipient mice were further retrovirally transduced with MSCVneo- FAS CDS (containing just the coding region of human FAS gene to avoid negative regulation of miR-196b) or MSCVneo through two rounds of spinoculation [26] . Then, the retrovirally transduced cells were plated into 35-mm Petri dishes in 1.1 ml of Methocult M3230 methylcellulose medium (Stem Cell Technologies Inc., Vancouver, Canada) containing 10 ng ml −1 each of murine recombinant IL-3, IL-6 and granulocyte-macrophage colony-stimulating factor, and 30 ng ml −1 of murine recombinant SCF (R&D Systems, Minneapolis, MN, USA), along with 1.0 mg ml −1 of G418 to select transduction-positive cells. Every 2×10 4 retrovirally transduced cells were plated in one dish. For each transduction, there were four duplicate dishes. Cultures were incubated at 37°C in a humidified atmosphere of 5% CO 2 in air. The colony cells were collected and washed after 6 days of culture, and then transplanted into sublethally irradiated (480 rads) 8- to 10-week-old B6.SJL (CD45.1) secondary recipient mice via tail vein injection, with 1×10 6 donor cells plus a radioprotective dose of whole BM cells (1x10 6 ; freshly harvested from a B6.SJL mouse) per secondary recipient mouse. The maintenance and end-point treatment of mice C57BL/6 (CD45.2) and B6.SJL (CD45.1) were purchased from the Jackson Lab (Bar Harbor, ME, USA) or Harlan Laboratories, Inc. (Indianapolis, IN, USA). Both male and female mice were used for the experiments. All laboratory mice were maintained in the animal facility at the University of Chicago. All experiments on mice in our research protocol were approved by Institutional Animal Care and Use Committee of the University of Chicago. PB cells were collected from the transplanted recipient mice monthly via tail bleeding and at any time that the mice showed signs of systemic illness to obtain the complete blood counts with white blood cell differentials and the blood smears for the presence of immature or abnormal haematopoietic cells. The degrees of engraftment were assessed by flow cytometry analysis of GFP and CD45.1 in PB. Leukaemic mice were euthanized by CO 2 inhalation if they showed signs of systemic illness, and some negative-control recipient mice were also killed at some time points (though they did not develop leukaemia) to collect specimens as conrtols for further analyses. The spleen, liver and thymus were weighed. Cells were obtained from the PB, BM, spleen and liver for flow cytometric analysis. Blood smear and BM cytospin slides were stained with Wright–Giemsa. Portions of the spleen and liver were collected for histolopathology and immunohistochemistry assays. Histolopathology and Immunohistochemistry Tissue samples were fixed in formalin, embedded in paraffin, sectioned and stained with haematoxylin and eosin. Cytospins were stained with Wright–Giemsa. In all experiments, immunostain was performed on 4 μm thick paraffin tissue sections of mouse spleens and livers on a Dako Autostainer (Dako, Carpinteria, CA, USA), using a monoclonal rabbit antibody anti-cleaved caspase-3 (Asp175) (5A1E; Cell Signalling Inc.) and rabbit EnVision-plus HRP (DAB)TM detection System (Dako). Briefly, following deparaffinization in xylene, hydration in alcohols and quenching the endogenous peroxidase in 3% hydrogen peroxide in methanol for 5 min and antigen retrieval in Target retrieval solution (Dako) in a water bath at 95°C for 40 min, sections were incubated with anti-cleaved caspase 3 (Asp175) at dilution 1:50 overnight at 4°C and subsequently transferred to the Dako Autostainer where they were incubated with detection system for 30 min. Peroxidase reaction was developed using DAB provided in the detection kit. Slides were counterstained with haematoxylin, dehydrated in alcohols and mounted in mounting medium (Sakura Finetek USA, Torrance, CA, USA). Immunoblotting Transiently transfected Hela, MONOMAC6 or mouse BM cells were harvested and lysed with RAPI buffer (Pierce, Rockford, IL, USA). Proteins from the lysate were fractionated by electrophoresis through 4–15% polyacrylamide gels (Bio-Rad, Hercules, CA, USA) and transferred to polyvinylidene fluoride membranes using Tris-Glycine Transfer buffer (Thermo Scientific, BufferRockford, IL, USA). After blocking with 5% milk, membranes were incubated with various antibodies and then processed for chemiluminescent detection with ECL Plus Western Blotting Detection Reagents (GE Healthcare, Piscataway, NJ, USA). Anti-HOXA9 or HoxA9 (Millipore, Billerica, MA, USA), Anti-MEIS1 or Meis1 (SDIX, Newark, DE, USA), Anti-FAS or Fas (Santa Cruz Biotechnology Inc., Santa Cruz, CA, USA), and anti-GAPDH (R&D Systems) were used for immunoblotting. Apoptosis assay MONOMAC6 or Jurkat cells were transfected with 100 nM of miR-196b mimic or Mimic Negative Control (Dharmacon Products, Lafayette, CO, USA) using Cell Line Nucleofector Kit V following program T-027 or X-001, respectively, with a nucleofector device (Amaxa Biosystems, Berlin, Germany). Cells were treated with purified Mouse Anti-Human CD95 (FAS) (EOS9.1, BD Pharmingen, San Jose, CA, USA) 48 h post transfection. Sixteen hours later, cells were analysed for Annexin V staining with Annexin V-FITC Apoptosis Detection Kit I (BD Pharmingen) by flow cytometry. How to cite this article: Li, Z. et al . miR-196b directly targets both HOXA9/MEIS1 oncogenes and FAS tumour suppressor in MLL -rearranged leukaemia. Nat. Commun. 3:688 doi: 10.1038/ncomms1681 (2012).